Neural crest cells organize the eye via TGF-β and canonical Wnt signalling In vertebrates, the lens and retina arise from different embryonic tissues raising the question of how they are aligned to form a functional eye. Neural crest cells are crucial for this process: in their absence, ectopic lenses develop far from the retina. Here we show, using the chick as a model system, that neural crest-derived transforming growth factor-βs activate both Smad3 and canonical Wnt signalling in the adjacent ectoderm to position the lens next to the retina. They do so by controlling Pax6 activity: although Smad3 may inhibit Pax6 protein function, its sustained downregulation requires transcriptional repression by Wnt-initiated β-catenin. We propose that the same neural crest-dependent signalling mechanism is used repeatedly to integrate different components of the eye and suggest a general role for the neural crest in coordinating central and peripheral parts of the sensory nervous system. In the vertebrate head, different components of the sensory nervous system develop from different embryonic tissues. For example, in the eye, the retina arises from the central nervous system, whereas the lens originates in the surface ectoderm [1] . An unresolved problem is how these components are aligned with each other to ensure normal structure and function. In the eye, it is generally accepted that the lens is induced by the optic vesicle (future retina) [1] , [2] , [3] , which would explain their alignment. However, we now know that lens induction begins before contact with the optic vesicle, and that much of the cranial ectoderm has intrinsic lens potential [4] , [5] , [6] . Therefore, lens potential must be actively suppressed in non-lens ectoderm. Our previous observations implicate neural crest cells (NCCs) in this process: NCC ablation in vivo causes ectopic lenses to develop, and NCCs repress lens specification in vitro [4] , [6] . Consistent with this, lens potential becomes gradually restricted during NCC migration [4] , [5] , [7] and NCCs invade most areas of the head, but never reach the future lens because the optic vesicle functions as a physical barrier [8] , [9] . Thus, NCCs inhibit lens development except in the vicinity of the retina, ensuring the alignment of peripheral (lens) and central (retina) components of the eye. However, the signals involved are unknown. Here we show that NCC-derived members of the transforming growth factor (TGF)-β subfamily activate both Smad3 and canonical Wnt signalling in the non-lens ectoderm. In the lens territory, both pathways prevent lens formation; however, their inhibition prevents lens suppression by NCCs. Thus, Smad3-mediated TGF-β and canonical Wnt signalling cooperate to restrict lens potential to the ectoderm overlying the retina, and thus have a critical role in the formation of a functional eye. TGF-β signalling inhibits lens specification The transcription factor Pax6 has a key role in eye development and is required for lens formation; it activates its own transcription as well as that of other lens-specific genes [10] , [11] , [12] , [13] , [14] . However, in vitro its autoregulation can be inhibited at the protein level by binding to phosphorylated Smad3 (pSmad3) after TGF-β stimulation [15] , implicating this as a candidate pathway for lens restriction. We found that multiple TGF-β ligands are expressed in migrating NCCs, but are absent from the lens, these included TGF-β1 , Activin-βA and Activin-βB ( Supplementary Fig. S1 ). Following contact with migrating NCCs, the adjacent non-lens ectoderm received TGF-β signals as shown by the presence of pSmad3, whereas lens ectoderm, which was protected from infiltrating NCCs by the optic vesicle, was pSmad3-negative ( Supplementary Fig. S2 ). Thus, members of the TGF-β subfamily, which signal through Smad2 and Smad3 (hereafter referred to as TGF-β for simplicity), are expressed in NCCs, and only non-lens ectoderm activates this pathway. To assess whether activated Smad3 suppresses lens fate in vivo, we electroporated constitutively active Smad3 (ref. 16 ) into the presumptive lens ectoderm (PLE). Although control green fluorescent protein-expressing cells were incorporated into the lens and express the lens marker δ-crystallin ( Fig. 1a–c ; 3/3 lenses), constitutively active Smad3-expressing cells were excluded from the lens and did not express δ-crystallin ( Fig. 1d–f ; 0/5 lenses). Together, the above results suggest that TGF-βs prevent lens formation at inappropriate positions. 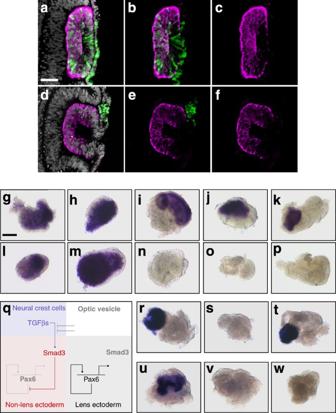Figure 1: TGF-β represses lens formation. (a–c) Presumptive lens ectoderm (PLE) was electroporated with expression vector encoding green fluorescent protein (GFP): (a) GFP-expressing cells (green) counterstained for δ-crystallin (magenta) and cell nuclei (grey); (b) GFP and δ-crystallin staining only; (c) δ-crystallin staining only. (d–f) PLE was electroporated with expression vector encoding constitutively active Smad3+GFP: (d) GFP-expressing cells (green) counterstained for δ-crystallin (magenta) and cell nuclei (grey); (e) GFP and δ-crystallin staining only; (f) δ-crystallin staining only. (g–k) PLE explants were culturedin vitroand assayed for pre-placodal (Six1, Eya2) or lens (Pax6, L-Maf, δ-crystallin) gene expression: (g)Six1; (h)Eya2; (i)Pax6; (j)L-Maf; and (k)δ-crystallin. (l–p) PLE explants were cultured in the presence of Activin A and assayed for pre-placodal or lens gene expression: (l)Six1; (m)Eya2; (n)Pax6; (o)L-Maf; and (p)δ-crystallin. (q) Model for lens inhibition by TGF-β signalling. (r–t) PLE explants were cultured alone or in combination with Activin A or SB431542 and assayed forδ-crystallingene expression: (r) PLE alone; (s) PLE+Activin A; and (t) PLE+Activin A+SB431542. (u–w) PLE explants were cultured alone or in combination with neural crest cells (NCC) or SB431542 and assayed forδ-crystallingene expression: (u) PLE alone; (v) PLE+NCC; and (w) PLE+NCC+SB431542. Scale bars:a, 50 μm for panelsa–f, g, 50 μm for panelsg–p,r–w. Figure 1: TGF-β represses lens formation. ( a – c ) Presumptive lens ectoderm (PLE) was electroporated with expression vector encoding green fluorescent protein (GFP): ( a ) GFP-expressing cells (green) counterstained for δ-crystallin (magenta) and cell nuclei (grey); ( b ) GFP and δ-crystallin staining only; ( c ) δ-crystallin staining only. ( d – f ) PLE was electroporated with expression vector encoding constitutively active Smad3+GFP: ( d ) GFP-expressing cells (green) counterstained for δ-crystallin (magenta) and cell nuclei (grey); ( e ) GFP and δ-crystallin staining only; ( f ) δ-crystallin staining only. ( g – k ) PLE explants were cultured in vitro and assayed for pre-placodal ( Six1, Eya2 ) or lens ( Pax6, L-Maf, δ-crystallin ) gene expression: ( g ) Six1 ; ( h ) Eya2 ; ( i ) Pax6 ; ( j ) L-Maf ; and ( k ) δ-crystallin . ( l – p ) PLE explants were cultured in the presence of Activin A and assayed for pre-placodal or lens gene expression: ( l ) Six1 ; ( m ) Eya2 ; ( n ) Pax6 ; ( o ) L-Maf ; and ( p ) δ-crystallin . ( q ) Model for lens inhibition by TGF-β signalling. ( r–t ) PLE explants were cultured alone or in combination with Activin A or SB431542 and assayed for δ-crystallin gene expression: ( r ) PLE alone; ( s ) PLE+Activin A; and ( t ) PLE+Activin A+SB431542. ( u – w ) PLE explants were cultured alone or in combination with neural crest cells (NCC) or SB431542 and assayed for δ-crystallin gene expression: ( u ) PLE alone; ( v ) PLE+NCC; and ( w ) PLE+NCC+SB431542. Scale bars: a , 50 μm for panels a – f, g , 50 μm for panels g – p , r – w . Full size image To study this further, we used an explant system that recapitulates endogenous lens development: pre-placodal gene expression ( Six1 , Eya2 ; Fig. 1g,h ; see Table 1 for numbers of all explant experiments) preceded the expression of Pax6 , L-Maf and δ-crystallin ( Fig. 1i–k ), each of which labels a distinct phase of lens formation. This allowed us to determine the stage at which TGF-β/Smad3 function to inhibit lens development. Culture of explants in Activin A did not affect the expression of early pre-placodal genes ( Fig. 1l,m ), but did prevent the expression of the later lens-specific markers ( Fig. 1n–p ). In cells in which lens markers were repressed, markers for other sensory structures were not induced ( Table 1 ; Pax3 + trigeminal, Pax2 + otic or FoxG1 + olfactory placodes), suggesting that Activin A maintains pre-placodal cells in an undifferentiated progenitor state, as shown for other cell types [17] , [18] . Thus, activation of TGF-β signalling prevents the acquisition of lens fate in vivo and in vitro and is likely to function by regulating Pax6. We propose that NCC-derived TGF-βs activate Smad3 in the overlying surface ectoderm, which may in turn sequester Pax6 protein [15] to prevent activation of downstream targets and lens formation ( Fig. 1q ). Table 1 Summary of in vitro experiments. Full size table Wnt signalling is required for lens repression by NCCs If TGF-β signalling alone is responsible for positioning the lens, inhibition of this pathway should rescue lens development in the presence of NCCs. To test this, we made use of the TGF-β receptor inhibitor SB431542 (SB) [19] . When cultured with both Activin A and SB, presumptive lens explants retained δ-crystallin expression, in contrast to treatment with Activin A alone ( Fig. 1r–t ). However, SB was unable to restore lens marker expression in the presence of presumptive NCCs ( Fig. 1u–w ), suggesting that, although TGF-β signalling is sufficient for lens inhibition, other signals must be involved. In mouse, canonical Wnt signalling suppresses lens development [20] . Consistent with this, we found that overexpression of constitutively active β-catenin in PLE prevented the expression of δ-crystallin. Although 83% of control cells were δ-crystallin + (66/87 cells in three lenses; Fig. 2a–c ), this was reduced to 35% when canonical Wnt signalling was activated (27/77 cells in five lenses; Fig. 2d–j ). Interestingly, similar to caSmad3-expressing cells ( Fig. 1d–f ), those carrying β-catenin were excluded from the lens over time: after 24 h β-catenin + /δ-crystallin − cells were found in the lens placode ( Fig. 2d–f ), but were mostly absent from the lens after 48 h ( Fig. 2g–i ). If Wnt signalling is involved in the residual lens-repressing activity of NCCs, Wnt inhibition should rescue lens development in the presence of NCCs. To test this, we cocultured NCCs and PLE with the Wnt antagonist N-Fz8. Indeed, inhibition of Wnt signalling rescued δ-crystallin expression ( Fig. 2k–m ), suggesting that Wnt is required for lens repression by NCCs and suppresses lens formation through β-catenin ( Fig. 2n ). 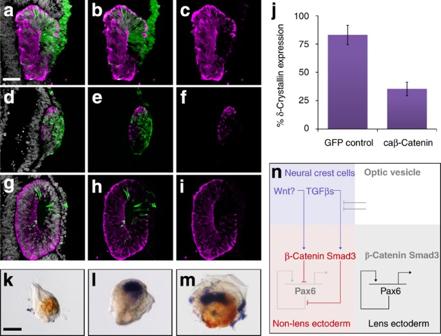Figure 2: β-Catenin inhibits lens formation, and Wnt signalling is required for lens repression by NCCs. (a–c). Presumptive lens ectoderm (PLE) was electroporated with expression vector encoding green fluorescent protein (GFP) and embryos were cultured for 48 h. (a) GFP-expressing cells (green) were stained for δ-crystallin protein (magenta) and cell nuclei (grey); (b) GFP and δ-crystallin staining only; (c) δ-crystallin staining only. (d–i) PLE was electroporated with caβ-catenin+GFP and embryos were cultured for 24 or 48 h. (d–f) Twenty-four hours: (d) GFP-expressing cells (green) were stained for δ-crystallin protein (magenta) and cell nuclei (grey); (e) GFP and δ-crystallin staining only; (f) δ-crystallin staining only. (g–i) Forty-eight hours: (g) GFP-expressing cells (green) were stained for δ-crystallin protein (magenta) and cell nuclei (grey); (h) GFP and δ-crystallin staining only; (i) δ-crystallin staining only. (j) Mean proportion of GFP+electroporated cells within the lens that also express δ-crystallin protein. GFP control:n=3 lenses; 66 of 87 electroporated cells express δ-crystallin. caβ-catenin:n=5 lenses; 27 of 77 electroporated cells δ-crystallin. Error bars: ±1 s.d. (k–m) PLE explants were cultured alone or in combination with neural crest cells (NCCs) or N-Fz8 and assayed for lens (δ-crystallin; brown) and NCC (CRABP1; blue) gene expression: (k) PLE alone; (l) PLE+NCC; (m) PLE+NCC+N-Fz8. (n) Model for lens inhibition by TGF-β and canonical Wnt signalling. Scale bars:a, 50 μm for panelsa–i;k, 50 μm for panelsk–m. Figure 2: β-Catenin inhibits lens formation, and Wnt signalling is required for lens repression by NCCs. ( a – c ). Presumptive lens ectoderm (PLE) was electroporated with expression vector encoding green fluorescent protein (GFP) and embryos were cultured for 48 h. ( a ) GFP-expressing cells (green) were stained for δ-crystallin protein (magenta) and cell nuclei (grey); ( b ) GFP and δ-crystallin staining only; ( c ) δ-crystallin staining only. ( d – i ) PLE was electroporated with caβ-catenin+GFP and embryos were cultured for 24 or 48 h. ( d – f ) Twenty-four hours: ( d ) GFP-expressing cells (green) were stained for δ-crystallin protein (magenta) and cell nuclei (grey); ( e ) GFP and δ-crystallin staining only; ( f ) δ-crystallin staining only. ( g – i ) Forty-eight hours: ( g ) GFP-expressing cells (green) were stained for δ-crystallin protein (magenta) and cell nuclei (grey); ( h ) GFP and δ-crystallin staining only; ( i ) δ-crystallin staining only. ( j ) Mean proportion of GFP + electroporated cells within the lens that also express δ-crystallin protein. GFP control: n =3 lenses; 66 of 87 electroporated cells express δ-crystallin. caβ-catenin: n =5 lenses; 27 of 77 electroporated cells δ-crystallin. Error bars: ±1 s.d. ( k – m ) PLE explants were cultured alone or in combination with neural crest cells (NCCs) or N-Fz8 and assayed for lens ( δ-crystallin ; brown) and NCC ( CRABP1 ; blue) gene expression: ( k ) PLE alone; ( l ) PLE+NCC; ( m ) PLE+NCC+N-Fz8. ( n ) Model for lens inhibition by TGF-β and canonical Wnt signalling. Scale bars: a , 50 μm for panels a – i ; k , 50 μm for panels k – m . Full size image Wnt represses lens fate downstream of NCC-derived TGF-βs In a survey of Wnt expression, we did not find any Wnt transcripts present in migrating NCCs. However, we did find a strong correlation between NCC migration and Wnt2b expression in the ectoderm: following contact with migrating NCCs, Wnt2b began to be expressed in the neighbouring ectoderm but remained absent from the prospective lens territory ( Fig. 3a–c ). The highest levels of Axin2 expression (a read-out of canonical Wnt activity) were present in ectoderm that had been in contact with NCCs for longest duration ( Fig. 3d,e , arrowheads; compare midbrain and forebrain levels). These observations suggest that NCCs initiate Wnt2b expression in the ectoderm in which lens formation is normally inhibited. Indeed, migratory NCCs strongly induced Wnt2b in presumptive lens explants, which normally do not express the transcript ( Fig. 3f,g ), suggesting that TGF-β may be the NCC signal responsible for ectodermal Wnt2b. Indeed, in vitro , Wnt2b induction by NCCs failed when TGF-β signalling was inhibited ( Fig. 3h ), whereas Activin A strongly induced Wnt2b in presumptive lens explants ( Fig. 3i,j ). Similarly, in vivo , ectodermal Wnt2b expression depended on TGF-β signalling from NCCs: NCC ablation ( Fig. 3k,l ) and misexpression of the inhibitory Smad7 ( Fig. 3m,n ; Smad7: 2/6 Wnt2b + , green fluorescent protein: 5/5 Wnt2b + ) caused downregulation of Wnt2b transcripts in the non-lens ectoderm. Together, these results show that TGF-β signalling from NCCs induces Wnt2b expression in the non-lens ectoderm. 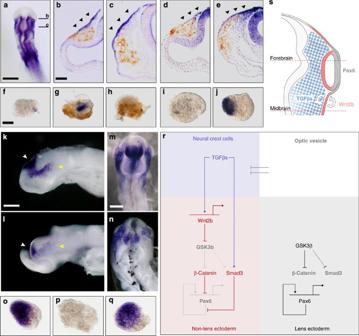Figure 3: Wnt mediates lens repression by NCCs and TGF-β. (a–c)Wnt2b(blue) gene expression during neural crest cell (NCC) migration: (a) Whole-mount embryo showing the forebrain section used in panelband the midbrains section used in panelc. (b) Forebrain level section stained forWnt2b; (c) midbrain level section stained forWnt2b. (d) Forebrain level section stained forAxin2gene expression (blue). (e) Midbrain level section showingAxin2expression. All sections are immunostained for NCC-specific HNK1 (brown). Arrowheads indicate gene expression in non-lens ectoderm. (f–h) Presumtive lens ectoderm (PLE) explants were cultured alone or in combination with NCC or SB431542 and assayed forWnt2bgene expression (blue) and HNK1 (brown): (f) PLE alone; (g) PLE+NCC; (h) PLE+NCC+SB431542. (i,j) PLE explants were cultured alone or with Activin A and assayed forWnt2bgene expression: (i) PLE alone; (j) PLE+Activin A. (k,l)Wnt2bgene expression (blue) followingin ovoablation of premigratory NCCs: (k) control embryo; (l) NCC ablated embryo. CompareWnt2bexpression in the brain (white arrowheads) with non-lens surface ectoderm (yellow arrowheads). (m,n)Wnt2bgene expression (blue) followingin ovoelectroporation of expression vectors encoding green fluorescent protein (GFP) or Smad7+GFP: (m) GFP; (n) Smad7+GFP. (o–q) PLE explants were cultured alone or in combination with Activin A or N-Fz8 and assayed forPax6gene expression (blue): (o) PLE alone; (p) PLE+Activin A; (q) PLE+Activin A+N-Fz8. (r) Proposed molecular model to explain TGF-β- and Wnt-mediated lens restriction. Broken lines: interactions inferred from the literature. (s) Proposed embryological model summarizing how NCCs organize the eye: NCCs (blue) secrete TGF-βs, which signal to the non-lens ectoderm and dorsal optic vesicle. As a consequence,Wnt2b(red) is induced, and together they repress lens formation in the non-lens ectoderm. This leads to the alignment ofPax6expression in the future lens and neural retina (grey). Scale bars:a, 500 μm;b, 50 μm for panelsb–e;f, 50 μm for panelsf–j,o–q;k, 250 μm for panelsk,l;m, 250 μm for panelsm,n. Figure 3: Wnt mediates lens repression by NCCs and TGF-β. ( a – c ) Wnt2b (blue) gene expression during neural crest cell (NCC) migration: ( a ) Whole-mount embryo showing the forebrain section used in panel b and the midbrains section used in panel c . ( b ) Forebrain level section stained for Wnt2b ; ( c ) midbrain level section stained for Wnt2b . ( d ) Forebrain level section stained for Axin2 gene expression (blue). ( e ) Midbrain level section showing Axin2 expression. All sections are immunostained for NCC-specific HNK1 (brown). Arrowheads indicate gene expression in non-lens ectoderm. ( f – h ) Presumtive lens ectoderm (PLE) explants were cultured alone or in combination with NCC or SB431542 and assayed for Wnt2b gene expression (blue) and HNK1 (brown): ( f ) PLE alone; ( g ) PLE+NCC; ( h ) PLE+NCC+SB431542. ( i , j ) PLE explants were cultured alone or with Activin A and assayed for Wnt2b gene expression: ( i ) PLE alone; ( j ) PLE+Activin A. ( k , l ) Wnt2b gene expression (blue) following in ovo ablation of premigratory NCCs: ( k ) control embryo; ( l ) NCC ablated embryo. Compare Wnt2b expression in the brain (white arrowheads) with non-lens surface ectoderm (yellow arrowheads). ( m , n ) Wnt2b gene expression (blue) following in ovo electroporation of expression vectors encoding green fluorescent protein (GFP) or Smad7+GFP: ( m ) GFP; ( n ) Smad7+GFP. ( o – q ) PLE explants were cultured alone or in combination with Activin A or N-Fz8 and assayed for Pax6 gene expression (blue): ( o ) PLE alone; ( p ) PLE+Activin A; ( q ) PLE+Activin A+N-Fz8. ( r ) Proposed molecular model to explain TGF-β- and Wnt-mediated lens restriction. Broken lines: interactions inferred from the literature. ( s ) Proposed embryological model summarizing how NCCs organize the eye: NCCs (blue) secrete TGF-βs, which signal to the non-lens ectoderm and dorsal optic vesicle. As a consequence, Wnt2b (red) is induced, and together they repress lens formation in the non-lens ectoderm. This leads to the alignment of Pax6 expression in the future lens and neural retina (grey). Scale bars: a , 500 μm; b , 50 μm for panels b – e ; f , 50 μm for panels f – j , o – q ; k , 250 μm for panels k , l ; m , 250 μm for panels m , n . Full size image The above findings suggest that the lens-repressing activity of TGF-β is mediated by Wnts. In the presence of Activin A, presumptive lens explants lose Pax6 transcripts ( Figs 1i,n and 3o,p ). However, when Wnt was simultaneously inhibited by N-Fz8, Pax6 expression was restored ( Fig. 3q ) demonstrating that lens suppression by TGF-β depends on active Wnt signalling. Together, these findings support a model in which NCC-derived TGF-βs initiate both Smad3 and canonical Wnt signalling to suppress lens fate in non-lens ectoderm ( Fig. 3r,s ). The formation of functional organs requires the integration of tissues with different embryonic origins; this is particularly evident in the vertebrate head in which peripheral components of sense organs or sensory ganglia must be perfectly aligned with their central counterparts to ensure normal function. Here we reveal the signalling network that controls this process in the vertebrate eye, in which the retina arises from the central nervous system and the lens from the surface ectoderm. Initial widespread lens potential [4] , [5] , [6] , [7] is gradually restricted to the ectoderm next to the retina through complex interactions of TGF-β and Wnt signalling ( Fig. 3r,s ). Migrating NCCs secrete TGF-βs, which in turn activate Smad3 and canonical Wnt signalling in the adjacent non-lens ectoderm. Although our studies implicate Wnt2b as the source of Wnt activity, it is possible that other, yet to be identified, ligands have a role. We propose that, to position the lens, TGF-βs initiate a 'double assurance' mechanism to regulate Pax6 function and transcription. Although pSmad3 may sequester Pax6 protein to inhibit its function as a transcriptional activator [15] , TGF-βs also function indirectly by inducing Wnt2b . In turn, Wnt2b may repress Pax6 transcription directly through β-catenin/TCF. Although generally thought to be a transcriptional activator, new evidence suggests that this complex can also directly repress transcription [21] , [22] . In support of this idea, the exon 1 enhancer of Pax6 [23] contains two conserved putative TCF-binding sites. The importance of β-catenin function in lens repression is also evident from studies in mouse, in which loss of β-catenin in the periocular ectoderm leads to the formation of small lentoids and rescues lens formation in Rx-deficient mice [20] , [24] . Thus, β-catenin has a critical role in preventing lens formation in inappropriate positions. In addition, high levels of pSmad3 in the non-lens ectoderm may depend on a Wnt2b-mediated feed-forward loop: canonical Wnt signalling not only stabilizes β-catenin but also Smad3 through inhibition of GSK3β [25] , [26] , [27] , suggesting that sustained TGF-β signalling is required to activate Smad3. Accordingly, pSmad3 stabilization directly correlates with high levels of canonical Wnt signalling induced by prolonged exposure to NCC-derived TGF-β (compare midbrain and forebrain levels in Supplementary Fig. S2 and Fig. 3d,e ). In contrast, Wnt signalling is absent in the future lens, partially because of the expression of Wnt antagonists [20] , [28] , and active GSK3β may mediate the degradation of both β-catenin and Smad3 (refs 25 , 26 , 27 ). Consequently, Pax6 remains expressed and initiates downstream lens specification. Thus, Wnt-dependent Smad3 and β-catenin signalling may provide a robust switch between lens and non-lens fate. Interestingly, the same signals may also pattern the optic vesicle; specification of pigment epithelium depends on head mesenchyme-derived TGF-βs, which in turn repress retinal fate [29] . Although Wnt2b is expressed in the pigment epithelium, its role in repressing retinal Pax6 has not been explored. Thus, Wnt and TGF-β signalling may be used repeatedly to organize different components of the eye. Our findings also highlight the fact that NCCs are crucial to ensure that central and peripheral parts of the eye become aligned in development: they prevent lens formation except next to the optic vesicle [4] , [5] , [6] . The optic vesicle itself seems to have a dual role providing lens-promoting signals [1] , [30] , [31] and functioning as a physical barrier to prevent apposition of NCCs and lens tissue. Like in chick, NCCs in humans are never in contact with the lens [9] , whereas in mouse they initially underlie the lens territory, but are subsequently displaced by the optic vesicle. This may explain why lens specification in mouse occurs only after optic vesicle contact [30] and why lens formation fails in mouse mutants that lack the optic vesicle [24] , [32] , [33] . In summary, NCCs emerge as key organizers of the vertebrate eye by contributing to the alignment of lens and retina and by patterning the optic vesicle. In addition, they have previously been implicated in coordinating the central (though not peripheral) projections from epibranchial placode-derived sensory ganglia [34] , [35] . It is therefore possible that one crucial function of NCCs lies in the integration of sensory structures, ensuring functional convergence of distinct embryonic components. The coemergence of both cell populations [36] may have offered a distinct advantage by enabling a diversity of complex sense organs to evolve in the vertebrate head. Embryo manipulation All experiments were performed in accordance with relevant guidelines and regulations of King's College London. Fertile hens' eggs (Henry Stewart) were incubated at 38 °C to collect embryos between stages 8 and 10 (HH: Hamburger and Hamilton [37] ). NCCs were ablated in ovo from HH8 embryos [4] ; using tungsten needles, the neural folds were removed bilaterally from posterior forebrain to anterior hindbrain levels. For in ovo electroporations [38] , plasmid DNA (2 μg ml −1 ) was injected between the vitelline membrane and the surface ectoderm; four 50-ms pulses of 7 V each were used at an interval of 1 s to transfect the surface ectoderm posterior to the lens or the PLE of HH8 embryos. The following constructs were used for electroporation: caβ-catenin [39] , Smad7 (ref. 40 ) and caSmad3 (ref. 41 ). Explant cultures For explant cultures, PLE was dissected from HH8 embryos and freed from underlying mesoderm using 0.01% dispase and tungsten needles [4] . For NCC cocultures, PLEs were cultured with dorsal neural folds isolated from HH8 embryos at midbrain and posterior forebrain levels, which give rise to migrating NCCs during the culture period. To demonstrate TGF-β-dependent Wnt2b induction, migrating NCCs dorsal to the optic vesicle or lateral to the midbrain were dissected from HH12–13 embryos using tungsten needles and 0.01% dispase [4] . All explants were placed on ice until use. Explants were cultured in 199 medium (Sigma), supplemented with N 2 (Invitrogen), NaHCO 3 (11 g l −1 ) and antibiotics. Collagen gels and culture media were supplemented with the following factors as required: 100-ng ml −1 Activin A (R&D Systems), 500-ng ml −1 N-Frz-8 (R&D Systems), 10-μM SB431542/0.1% dimethylsulphoxide (Tocris) or 0.1% dimethylsulphoxide only (controls). In situ hybridization Embryos and explants were processed for in situ hybridization [42] using DIG-labelled antisense probes for Six1 [39] , Eya2 [43] , Pax6 [44] , L- Maf [45] , δ-crystallin [4] , Wnt2b (a gift from Susan Chapman), CRABP1 (a gift from Anthony Graham), TGFβ1 , ActivinβA , ActivinβB [46] and Nodal [47] . After incubation with anti-DIG antibodies (Roche) and washing, 4.5-μl nitroblue tetrazolium (50 mg ml −1 ) and 3.5-μl 5-bromo-4-chloro-3-indolyl phosphate (50 mg ml −1 ) per 1.5-ml developing solution were used for colour development. Images were acquired using an AxioCam and Axiovision software; all explants were photographed at the same magnification (×90) on an Olympus SX12. Immunohistochemistry Embryos were collected in PBS and fixed for 1 h at room temperature in 3.7% formaldehyde/PBS, supplemented with 1:1000 Phosphatase Inhibitor Cocktail 2 (Sigma). Immunocytochemistry was performed on cryosections [4] , using HNK-1 antibody (1:10), antibodies against pSmad3 (Cell Signalling Technology; 1:100) and δ-crystallin (a gift from Joram Piatigorsky; 1:2,500) and Alexa-coupled secondary antibodies (Invitrogen; 1:1000). All antibodies were diluted in blocking buffer (5% goat serum, 0.1% Triton X-100 in PBS). Sections were photographed using a Leica LSM confocal microscope. How to cite this article: Grocott, T. et al . Neural crest cells organize the eye via TGF-β and canonical Wnt signalling. Nat. Commun. 2:265 doi: 10.1038/ncomms1269 (2011).